Sub-diffractional volume-confined polaritons in the natural hyperbolic material hexagonal boron nitride Strongly anisotropic media, where the principal components of the dielectric tensor have opposite signs, are called hyperbolic. Such materials exhibit unique nanophotonic properties enabled by the highly directional propagation of slow-light modes localized at deeply sub-diffractional length scales. While artificial hyperbolic metamaterials have been demonstrated, they suffer from high plasmonic losses and require complex nanofabrication, which in turn induces size-dependent limitations on optical confinement. The low-loss, mid-infrared, natural hyperbolic material hexagonal boron nitride is an attractive alternative. Here we report on three-dimensionally confined ‘hyperbolic polaritons’ in boron nitride nanocones that support four series (up to the seventh order) modes in two spectral bands. The resonant modes obey the predicted aspect ratio dependence and exhibit high-quality factors ( Q up to 283) in the strong confinement regime (up to λ /86). These observations assert hexagonal boron nitride as a promising platform for studying novel regimes of light–matter interactions and nanophotonic device engineering. Confining radiation to length scales much shorter than the diffraction limit at a given free-space wavelength λ ( ω ) is the primary focus of nanophotonics. There are two established approaches to this goal. One relies on materials of high positive permittivity Re ε ( ω ), wherein photons can be confined to the volume of the nanostructure [1] , [2] , [3] . This allows one to achieve a high optical density of states; however, the confinement length scale cannot be smaller than , which is a modest effect at visible frequencies. The other route utilizes materials where Re ε ( ω ) is negative, for example, metals at a frequency ω below the plasma frequency, ω p (ref. 4 ). In such media, electromagnetic energy can be localized in the form of surface plasmons. In the absence of losses, Im ε ( ω )→0, the smallest wavelength of such surface excitations is limited only by the microscopic structure, for example, the dimension a of the atomic unit cell. However, in reality, electronic losses are significant [5] , [6] , [7] , making this ultimate limit difficult to attain. Hyperbolic materials (HMs) [8] , [9] , [10] , [11] , [12] , [13] , [14] , [15] , whose permittivity tensor possesses both positive and negative principal components, have been proposed to enable novel functionalities that combine the advantages of strong confinement with full utilization of the material volume. The modes that make this possible are the high-momenta extraordinary rays—hyperbolic polaritons (HPs). The HP isofrequency surfaces are open hyperboloids, of either Type I ( Fig. 1a , left) if Re ε z <0, Re ε t >0 or Type II ( Fig. 1a , right) if Re ε z >0, Re ε t <0. (Here and below we assume a uniaxial anisotropy and label the tangential and axial components by t and z , respectively.) 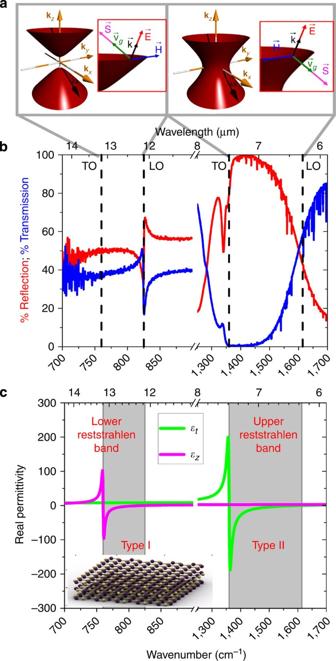Figure 1: Behaviour of the natural HM hBN. (a) Schematic isofrequency surfaces for a Type I (left) and II (right) hyperbolic media. The arrows in the insets indicate the directions of the electric (E) and magnetic (H) fields, the Poynting vector (S), the momentum (k) and the group velocity (vg) of the HP modes. The isofrequency contours each correspond to different spectral regions of hBN. (b) FTIR reflection (red curve) and transmission (blue curve) spectra of a 900-nm thick hBN flake exfoliated onto a 500-μm thick BaF2substrate. The frequencies of the TO and LO optic phonons of hBN in the axial and tangential directions are shown by the vertical dashed lines. (c) Derived real parts of the permittivity tensor components of hBN. The Type I lower and II upper Reststrahlen bands are shaded. A schematic of the hBN crystal structure is presented in the inset. At large k , the hyperboloids of both types can be approximated by cones, Figure 1: Behaviour of the natural HM hBN. ( a ) Schematic isofrequency surfaces for a Type I (left) and II (right) hyperbolic media. The arrows in the insets indicate the directions of the electric (E) and magnetic (H) fields, the Poynting vector (S), the momentum (k) and the group velocity (v g ) of the HP modes. The isofrequency contours each correspond to different spectral regions of hBN. ( b ) FTIR reflection (red curve) and transmission (blue curve) spectra of a 900-nm thick hBN flake exfoliated onto a 500-μm thick BaF 2 substrate. The frequencies of the TO and LO optic phonons of hBN in the axial and tangential directions are shown by the vertical dashed lines. ( c ) Derived real parts of the permittivity tensor components of hBN. The Type I lower and II upper Reststrahlen bands are shaded. A schematic of the hBN crystal structure is presented in the inset. Full size image In this approximation, the allowed directions for the momentum or the phase velocity of the HPs are restricted to the angle with respect to the optical axis [16] . HMs stand in a stark contrast to conventional media with positive Re ε z and Re ε t (for example, the free space) where the magnitude rather than direction of is restricted, resulting in a more familiar closed isofrequency surface (for example, a sphere). The field polarization of the HP is also unusual. As shown in the insets of Fig. 1a , the electric field is parallel to the momentum, while the magnetic field is azimuthal. As a result, the Poynting vector is orthogonal to the phase velocity (parallel to in Fig. 1a ). Both and the group velocity have a fixed angle with respect to the z axis, for example, for the k z >0 cone. This angle, which defines the propagation direction of the HPs, will play an important role in the later discussion. The rigid directionality of HPs serves as a basis for their proposed applications in super-resolution imaging and nanolithography [12] , [13] . The scale invariance of equation (1) implies that the HP modes can be localized inside extremely small volumes. Recent advances in the growth and exfoliation of high-quality hexagonal boron nitride (hBN), a natural HM, enabled the initial test of this prediction in experiments done on slabs of hBN thinned down to a thickness as small as d z ~1 nm. These scanning near-field optical studies [17] were able to detect the HP modes with momenta . Higher-order modes with , l =2, 3, … were also predicted but not yet observed. These experiments demonstrated an ultra-high confinement, ~ λ /10 4 albeit only along the axial ( z ) direction. Experimental demonstrations of HPs strongly confined in all three directions have to this point been limited to artificial metamaterials of the Type II variety built from alternating layers of Ag and Ge [18] . However, the smallest wavelength of HPs achievable in such structures is set by the size a of the repeated unit cell, below which the effective medium approximation fails [15] , [19] , [20] . This limits the use of hyperbolic metamaterials for truly nanoscale photonic applications. Indeed, the confinement reported did not exceed λ /12 in that work. In addition, the use of metallic layers that are plagued by considerable losses [6] , [21] caused the resonances to be rather broad (quality factors , where ω res and Δ ω res are the resonant frequency and linewidth) and the number of the modes observed [18] to be limited to just the first and in some cases second orders. Alternative approaches utilizing low-loss materials, such as those incorporating polar dielectrics supporting surface phonon polaritons (SPhPs) that are operational in the mid-infrared to THz spectral ranges [5] , rather than metal-based surface plasmons, can offer other potential improvements and in some cases additional functionality [22] , [23] , such as multi-frequency hyperlensing [23] . However, in all of these previously discussed hyperbolic metamaterials, the sign of the permittivity tensor was fixed by the geometry of the hybrid structure, resulting in either Type I or Type II behaviour for a given sample. This limits the design flexibility and makes it difficult to directly probe the physical differences between these two types of hyperbolic response. To fully explore the fundamental phenomena and applications of HM, it is desirable to work with material systems that possess low losses, have unit cells of nanoscale dimensions and feature both types of hyperbolic response. Here we report on experimental observations of HPs in hBN, a material satisfying all of these specifications. We detected the HP modes through optical reflection and transmission measurements performed on periodic arrays of conical hBN nanoparticles. These HP modes are manifested as resonances within two different mid-infrared spectral regions known as the lower and the upper Reststrahlen bands. We observed two distinct series of resonances per band (four in total). As many as seven modal orders in each series have been identified, consistent with the low optical losses of hBN, which are generic for SPhPs in polar dielectrics [5] , [24] , [25] . We have verified the fundamental hyperbolic dispersion (equation (1)) as the origin of the resonances by studying their dependence on polarization and the incident angle of the excitation beam, as well as on the size and shape of the nanocones, comparing these results with numerical and analytical calculations. In particular, the opposite dependence of the resonant frequency on the modal order (ascending versus descending in ω ) in the lower and upper Reststrahlen bands are the signatures of the Type I and Type II hyperbolic behaviour, respectively, and so they are realized simultaneously in this material. The observed modes possess record high-quality factors ( Q up to 283) (ref. 24 ) for sub-diffractional resonators and confinement ratios ( λ /86 in the smallest structures). These results identify hBN as a natural HM eminently suitable for exploring new fundamental physics and represents the first foray into creating natural HM [17] , [26] building blocks for mid-infrared nanophotonic devices [5] . 3D-confined HPs in hBN The mid-infrared hyperbolic response of hBN arises naturally from an extreme anisotropy of its optic phonon spectra. In general, the permittivity of a polar dielectric is negative inside its Reststrahlen band(s) and positive otherwise. The Reststrahlen bands are the spectral intervals between the longitudinal (LO) and transverse (TO) optic phonon frequencies and give rise to sub-diffraction, photonic confinement through SPhP stimulation [5] . In hBN, a layered van der Waals crystal [27] , the ab - and c axis-polarized phonons are widely separated in frequency so that the two Reststrahlen bands are non-overlapping in frequency. In experiments, they manifest themselves as high reflectivity (low transmission) intervals in the Fourier transform infrared (FTIR) spectra. An example is shown in Fig. 1b for a 900-nm-thick hBN flake on BaF 2 . The optical axis (our z axis) of the flake is the c axis of hBN ( Fig. 1c , inset). The plots of the derived permittivity components Re ε t >0 (green curve) and Re ε z (magenta curve) presented in Fig. 1c verify that Re ε z <0, Re ε t >0 in the lower band ( λ ≈12.1–13.2 μm) while Re ε t <0 Re ε z >0 in the upper ( λ ≈6.2–7.3 μm) band (shaded regions in Fig. 1c ). This means that the lower represents a Type I and the upper band a Type II hyperbolic response. To confine HPs in three dimensions to probe them in the far field, we used electron beam lithography and reactive ion etching to fabricate conical nanoresonators from hBN flakes of thickness 80–410 nm deposited on SiO 2 /Si, quartz or intrinsic silicon substrates. A scanning electron microscope image of a representative array and an individual nanocone are provided as an inset to Fig. 2b,c , respectively. The mid-infrared reflection spectra collected from a periodic 600-nm pitch array of hBN resonators of height d z =410 nm and diameter d t =375 nm on quartz are presented for near normal (red curve), ~25° off normal (green curve) and ~70° grazing incidence (blue curve) excitations (see schematic in Fig. 2a ). Here and below, d t stands for the diameter of a cylindrical resonator with the same height and volume as the truncated cone (see Supplementary Methods ). In the case of the grazing incidence measurements, p -polarized light was used to ensure that the axial modes were efficiently excited, while the near- and off-normal excitations were performed with unpolarized light to couple to both axial and tangential modes. The corresponding spectra are provided in Fig. 2a,b , respectively. They reveal distinct series of resonances within the two Reststrahlen bands. Invariably, the stronger series of resonances within each band is excited when the external electric field is parallel to the direction along which the permittivity is the most negative. The weaker modes are stimulated with the orthogonal polarization. For instance, within the lower band, the strongest response is observed with p -polarized, grazing incidence light (the blue curve in Fig. 2a ), while the second set of modes is preferentially observed at near-normal excitation (the red curve with asterisks in Fig. 2a ). The superposition of these resonances is observed at the off-normal excitation, resulting in Fano-like [28] , [29] lineshapes (the green curve in Fig. 2a ). Due to the inversion of the signs of the permittivity tensors along the principal axes within the two spectral regions, the incident angle and polarization required to excite the two sets of modes are reversed for the upper Reststrahlen band (for example, the stronger response is observed with near-normal and the weaker with p -polarized, grazing incidence excitation). Another conspicuous fact is that the two Reststrahlen bands exhibit opposite spectral trends. In both cases, full series of modes are observed, with each successive, reduced amplitude resonance corresponding to a higher modal order (as described below). The opposite spectral trends are clearly observed in the frequency shift for these higher-order resonances, which occur at larger ω in the lower, but at smaller ω in the upper Reststrahlen band. This behaviour is common to both the strong and weak resonance series in each band. 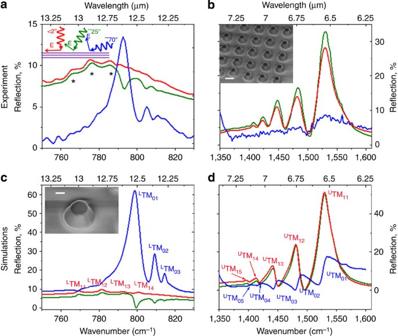Figure 2: HPs in hBN nanocones. FTIR reflection spectra of the (a) lower and (b) upper Reststrahlen bands collected from a periodic array (600 nm centre-to-centre pitch) of 375-nm diameter, 410-nm tall hBN conical nanoresonators. The spectra were collected using three different IR objectives giving rise to incident angles near normal (<2°, red curve), off-normal (~25°, green curve) and at near-grazing incidence (~70°, blue curve), with a schematic of these measurements provided as the inset ina. The weaker series of resonances observed in the lower Reststrahlen band are designated with ‘*’ as discussed in the text. For clarity, the near-grazing incidence spectra is offset by −4% ina. A scanning electron microscopic (SEM) image of a representative hBN nanoresonator array is provided as the inset inbwith the scale bar being 500 nm. (c,d) The reflection spectra calculated for the nanoresonator arrays ina,bfor both Reststrahlen bands using the finite-element method. The mode assignments are explained in the text and are defined using the notation, where TM defines the transverse magnetic nature of the mode,m, lare thezaxis angular momentum and orbital index, whileRdefines whether the modes are observed within the upper (‘U’) or lower (‘L’) Reststrahlen band. Inset: a SEM image of a single hBN nanoresonator with the scale bar being 200 nm. Figure 2: HPs in hBN nanocones. FTIR reflection spectra of the ( a ) lower and ( b ) upper Reststrahlen bands collected from a periodic array (600 nm centre-to-centre pitch) of 375-nm diameter, 410-nm tall hBN conical nanoresonators. The spectra were collected using three different IR objectives giving rise to incident angles near normal (<2°, red curve), off-normal (~25°, green curve) and at near-grazing incidence (~70°, blue curve), with a schematic of these measurements provided as the inset in a . The weaker series of resonances observed in the lower Reststrahlen band are designated with ‘*’ as discussed in the text. For clarity, the near-grazing incidence spectra is offset by −4% in a . A scanning electron microscopic (SEM) image of a representative hBN nanoresonator array is provided as the inset in b with the scale bar being 500 nm. ( c , d ) The reflection spectra calculated for the nanoresonator arrays in a , b for both Reststrahlen bands using the finite-element method. The mode assignments are explained in the text and are defined using the notation , where TM defines the transverse magnetic nature of the mode, m, l are the z axis angular momentum and orbital index, while R defines whether the modes are observed within the upper (‘U’) or lower (‘L’) Reststrahlen band. Inset: a SEM image of a single hBN nanoresonator with the scale bar being 200 nm. Full size image Altogether we studied and recorded resonance frequencies for 24 different samples. Each was a periodic array of hBN nanoresonators, but d z (height) and d t (width) were varied. Qualitatively, similar results were observed from all of the arrays (see Supplementary Figs 6–8 for more details); however, the positions of the resonant peaks were different for each sample. To test a possible scaling behaviour, we have plotted these frequencies as a function of the aspect ratio Remarkably, the entire data have been found to cluster along a set of well-defined smooth curves in such a plot, as shown in Fig. 3 , with each curve representing a different modal order. (The labelling of the modes in the figures is explained in the next section.) 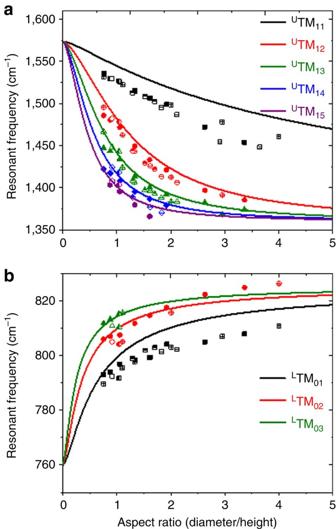Figure 3: Aspect ratio dependence of HP resonances. Analytical calculation of the aspect ratio dependence of the resonant frequencies of spheroidal nanoresonators in the (a) upper and (b) lower Reststrahlen bands. For simplicity, onlyandmodes are shown. The measured resonance frequencies for the fabricated hBN conical nanoresonators are provided by the various symbols. Different symbols refer to data obtained for arrays with different nanoresonator heights. In all, the data was collected from 24 different arrays of varying heights and diameters. Figure 3: Aspect ratio dependence of HP resonances. Analytical calculation of the aspect ratio dependence of the resonant frequencies of spheroidal nanoresonators in the ( a ) upper and ( b ) lower Reststrahlen bands. For simplicity, only and modes are shown. The measured resonance frequencies for the fabricated hBN conical nanoresonators are provided by the various symbols. Different symbols refer to data obtained for arrays with different nanoresonator heights. In all, the data was collected from 24 different arrays of varying heights and diameters. Full size image Theoretical analysis of hBN nanoresonators To investigate the physical origin of the observed resonances, we carried out numerical simulations of the reflectivity spectra. The results, shown in Fig. 2c,d , theoretically verify the existence of both the strong and weak series of resonances in each Reststrahlen band (four in total). The small discrepancies among the measured and calculated resonance frequencies may be attributed to slight irregularities in the shape of the actual nanoparticles compared with the idealized truncated cone used in the modelling. The incident polarization and angle requirements in the simulations are also consistent with those found in the experiments. Thus, the dominant resonance series within each band is excited when the external field is parallel to the negative permittivity direction. The opposite order of the frequency shifts in the two bands (increasing in the lower Reststrahlen versus decreasing in the upper Reststrahlen) is reproduced by the simulations as well. Further insight into the nature of the modes is provided by the electric field distribution inside the particles computed for the dominant resonances in the lower and upper bands, which are presented in Fig. 4a,b , respectively. In an effort to uncover the impact of hyperbolicity on the field distributions, concurrent calculations were performed for fictitious isotropic materials with permittivity equal to ε z ( Fig. 4c ) and ε t ( Fig. 4d ) of hBN. The isotropic response results in surface-confined distributions typical of surface plasmons [4] and surface phonon-polaritons [24] . In contrast, in the hyperbolic case, the field is volume confined, whereby the evanescent decay of the near-fields within the volume of the hyperbolic structures is not apparent, as demonstrated in Fig. 4a,b . In addition, the E -field distribution exhibits an intriguing ‘cross-hatch’ pattern, which is undoubtedly related to the directionality of the HP propagation. Indeed, the angle between the high-field crossing lines and the z axis is numerically close to the angle θ ( ω ) given by equation (2) [16] . These directional HP rays appear to be preferentially emitted by the top and bottom edges of the nanocones. The rays subsequently zigzag through the particle experiencing total internal reflections at the surface. The reason why these rays are predominantly launched at the edges is not completely clear, but we speculate it could be due to the generic tendency to find a singular field enhancement near sharp geometric features. The electric and magnetic field distributions for the principal and for several of the higher-order modes are presented in Fig. 5a–d . (The movies of the time-variation of these fields are provided in Supplementary Movies 1–4 .) The cross-hatch pattern in E is evident for the stronger resonance series both in the lower (70° incidence angle, Fig. 5a ) and upper (0° incidence angle, Fig. 5c ) Reststrahlen bands. For these surface plots, we selected the field components along the directions where they have the highest amplitude: parallel to the negative permittivity direction for the electric field and along the azimuthal y axis for the magnetic field. To show the magnetic field distribution due to the confined HP modes more clearly, we subtract the average H y that is largely due to the uniform illumination of the particle (the incident field plus its reflection off the underlying substrate). As mentioned above, the reduced amplitude resonances correspond to higher-order modes that are characterized by the progressively increasing number of the extrema (minima and maxima) of the electric and magnetic fields, as shown in Figs 5a – d , respectively. 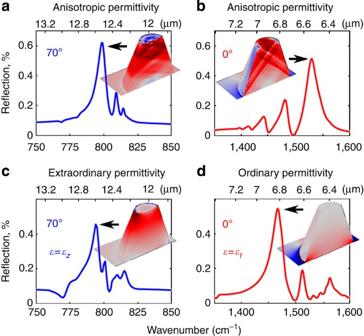Figure 4: Comparison of hyperbolic and isotropic behaviour for hBN. Simulated reflection spectra for the lower (a,c) and upper (b,d) Reststrahlen bands at 70 and 0° incident angles, respectively. (a,b) Case of a HM with anisotropic optical constants (top). (c) Same for a fictitious isotropic material with permittivityεt. (d) Same for a material with permittivityεz. The cross-sectional spatial distributions of |E| for the highest amplitude peak in each graph are provided as insets. Figure 4: Comparison of hyperbolic and isotropic behaviour for hBN. Simulated reflection spectra for the lower ( a , c ) and upper ( b , d ) Reststrahlen bands at 70 and 0° incident angles, respectively. ( a,b ) Case of a HM with anisotropic optical constants (top). ( c ) Same for a fictitious isotropic material with permittivity ε t . ( d ) Same for a material with permittivity ε z . The cross-sectional spatial distributions of | E | for the highest amplitude peak in each graph are provided as insets. 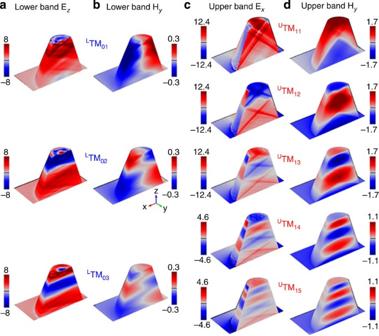Figure 5: Electromagnetic field simulations of Type I and II HPs in hBN nanocones. Simulated cross-sectional surface plots of the (a)Ezand (b)Hywithin the lower and (c)Exand (d)Hyfield components within the upper Reststrahlen bands of hBN for each of the resonant modes observed for the stronger series of resonances (Eparallel to the negative permittivity crystal axis). The incident angle was set to (a,b) 70° and (c,d) 0° to match the experiments. The assignment of the modes is discussed in the text. Full size image Figure 5: Electromagnetic field simulations of Type I and II HPs in hBN nanocones. Simulated cross-sectional surface plots of the ( a ) E z and ( b ) H y within the lower and ( c ) E x and ( d ) H y field components within the upper Reststrahlen bands of hBN for each of the resonant modes observed for the stronger series of resonances ( E parallel to the negative permittivity crystal axis). The incident angle was set to ( a , b ) 70° and ( c , d ) 0° to match the experiments. The assignment of the modes is discussed in the text. Full size image We have also compared numerically calculated spectra of arrays with those of isolated hBN nanocones. We concluded that the interparticle coupling in the arrays should be quite small for most of the samples studied, and so it is permissible to seek a more intuitive physical explanation of the observed spectra in terms of the mode structure of a single resonator. This is done in the next section where we address the polarization selection rules, the spectral shifts and the origin of the data collapse as a function of the aspect ratio. Historically, exact results available for certain regular shapes, for example, the celebrated Mie theory for the sphere played a major role in theoretical studies of light scattering by small particles [30] . It has been known for some time that the sphere and, more generally, spheroid admits an analytical solution for the case of arbitrary uniaxial anisotropy, including the hyperbolic regime [31] , [32] . We found this solution to be extremely helpful for the conceptual understanding of the present case of nanocone resonators, and so we briefly discuss it below. The eigenmodes of a spheroid with the symmetry axis parallel to the optical anisotropy axis can be labelled by three quantum numbers. The first, m =0, 1, … is the z axis angular momentum. The other two are the orbital index l = m , m +1, m +2, … and the radial index r =0, 1, …, r max (where 2 r max + m ≤ l ) that specify the number of nodes of the scalar potential Φ (related to the electric field by ) along the meridian and the radius. Coupling of these modes to far-field radiation is determined by the dipole selection rules. In particular, only m =0 and m =1 families are observable. They couple to photons polarized parallel and perpendicular to the z axis, respectively. In addition, modes of non-zero r would produce only weak resonances because of their small dipole moment. Below, we neglect them and suppress the radial index assuming it is equal to zero. The observable modes of the spheroid can therefore be denoted TM ml , where ‘TM’ (transverse magnetic) indicates that the magnetic field is orthogonal to the optical axis ( Fig. 1a insets). The dipole resonances l =1 are the dominant modes. They appear at frequencies satisfying the condition [30] , where L j ( A ) is the depolarization factor of the spheroid along the polarization direction j = z , t of the incident field. Equations for higher-order modes can be found in Supplementary Methods (see also the approximate equation (4) below). Because of the scale invariance of the problem, the resonant frequencies depend not on the absolute dimensions of the resonator but only on its aspect ratio A . For example, in the A →0 limit (needle-like particle), the dipole resonance conditions ε z ( ω )=−∞ for TM 01 and ε t ( ω )=−1 is for TM 11 generate the entire TM 0 l and TM 1 l series (the dominant series). In the opposite limit A →∞ (disk-like particle or a slab), the conditions to these series change to ε z ( ω )=0 and ε t ( ω )=−∞, respectively. (The permittivity of any physical system, and so the solutions ω = ω res − i Δ ω res of these equations, are complex. As usual, the imaginary parts represent the broadening and the real parts are the actual resonant frequencies.) Using the derived optical constants of hBN ( Fig. 1c and Supplementary Fig. 2a,b ) we plotted the dispersion curves of the spheroid as a function of the aspect ratio in Fig. 3 (computational details are provided in Supplementary Methods ), adding a left superscript (L or U) to the mode notation to discriminate the Reststrahlen band (lower or upper). In the lower band, the starting point A =0 of the curves is at the bottom of the band, ω TO, z =760 cm −1 . The mode frequencies monotonically increase toward ω LO, z =825 cm −1 . Both these extremal points and the trend can be understood from the fact that the depolarization factor L z monotonically increases from 0 to 1 as a function of A . In the upper band, the curves start at ω =1,575 cm −1 , somewhat red-shifted from the TO phonon frequency ( ω LO, t =1,614 cm −1 ), and monotonically decrease toward ω TO,t =1,370 cm −1 . It is readily apparent that experimental data (symbols in Fig. 3 ) exhibit the same qualitative dependence on the aspect ratio and are even quantitatively close to the theoretical dispersion plots. The agreement is impressive given the obvious difference in shape (truncated cones versus spheroids) and the effect of the substrate, which is disregarded in the theoretical calculations. As already mentioned, the resonance spectra are not only nominally independent of the absolute dimensions of the sub-diffractional particles, but ( Fig. 3 ) also indicate that a stronger statement is valid—that the spectra are also relatively insensitive to the fine details of the particle shape as well. Taken as a guiding principle, this permits us to use the same modal notations R TM ml for each of the resonances depicted in Figs 2 , 3 , 4 , 5 . This principle immediately explains the majority of our experimental observations. It elucidates the reason for the data collapse of the resonant frequencies for various sized nanostructures on a single aspect ratio trend for a given modal order. In other words, this describes how two arrays of hBN resonantors with large differences in size (for example, d z / d t =185/300 nm and d z / d t =340/550 nm) but the same aspect ratio ( A ~1.62) exhibit similar L TM 01 and U TM 11 resonance frequencies (799.5 and 1,506 cm −1 , respectively). It also clarifies why the number of observed resonance series in each band is exactly two (they correspond to m =0 and m =1) and why the polarization selection rule for the strongest resonances exists. Indeed, such resonances correspond to the l =1 dipole modes that get excited only by that electric field component j = t , z along which the permittivity is negative. A qualitative insight into the structure of the weaker resonance series is provided by the semiclassical method frequently used to analyse high-order optical modes l, m >>1 (for example, whispering-gallery modes) of dielectric resonators. In the semiclassical picture, the HPs propagate inside the nanoresonator as directional rays that experience total internal reflections at the boundaries. Depending on the shape of the particle, the mechanics of such rays can be either chaotic or regular [33] . In the spheroidal geometry we have the latter, in which case we have a simple quantization rule. It is basically the standing-wave conditions k z d z ~ l and k t d t ~ m imposed on the characteristic momenta k z and k t of the HP. We can combine these conditions with equations (1) and (2) to find the equation for the eigenfrequencies ω : The qualitative trends of the spectra can be understood without expressly solving equation (4). In the lower Reststrahlen band, the right-hand side of equation (4) is the increasing function of ω . Hence, if m and the aspect ratio are fixed, the resonance frequency should be higher for higher index l . In the upper Reststrahlen band, the right-hand side of equation (4) is a decreasing function, and so the modal order is opposite. This predicted inversion of these trends is in agreement with our observations ( Fig. 2 ). By a similar argument, the frequencies of high-order modes R TM ml should increase (decrease) as a function of the aspect ratio for R =L (U). The anomalous behaviour of the upper Reststrahlen band was also reported within Ag/Ge Type II hyperbolic metamaterial resonators [18] . Note that the spectral shifts have the same sign as the z component of the group velocity ν z =∂ ω /∂ k z of the HP. As shown by the green arrows in Fig. 1a left (right), ν z is positive (negative) in Type I (II) case. Extrapolated to the case m =1, equation (4) implies a simple rule regarding the discussed cross-hatch pattern of the electric field distribution. From elementary geometrical considerations, the total number of the ray intersections along the nanocone axis should be equal to N = A −1 tan θ ( ω ). In view of equation (4), this yields N ~ l / m = l , that is, the number of intersections is equal to the modal index. This approximate rule is in fact closely obeyed by all the m =1 modes shown in Fig. 5c . Although no such simple rule can be given for m =0, we may expect N > l in this case, which is also borne out by the simulations ( Fig. 5a ). Concluding this discussion, it is instructive to compare the figures-of-merit of our nanoresonators with those in literature. The modes observed here exhibit narrow linewidths and high-quality factors: Q tot =156–264 and 66–283, respectively, in the Type I lower and Type II upper Reststrahlen bands. These Q -factors are almost two orders of magnitude higher than Q tot ~ 4 reported for Type II hyperbolic metamaterial nanostructures [18] , and correspond to record values for sub-diffractional modes [24] , [34] , [35] . As the Q -factor defines the energy stored to energy loss rate, this can be inferred as a metric defining the resonator efficiency. These high-quality factors are also coupled with exceptional modal confinements as the size of our nanoresonators are 17–86 times smaller than the free-space wavelength in the z direction and 6–61 times smaller in the transverse direction. Such mode confinement factors are unprecedented in metal-based surface-plasmon nanostructures. For comparison, the highest confinement achieved for hyperbolic metamaterial structures was λ /12 (ref. 18 ) While similar confinements have been reported for plasmons in patterned graphene [36] , [37] , strong electronic losses limited the Q tot to values between 2.5 and 15. Such losses are fundamentally absent in hBN due to its polar dielectric nature [5] , [24] , [25] . In summary, this work constitutes the experimental observation of sub-diffractional guided waves confined in all three dimensions inside a natural HM. Compared with similar efforts in metamaterials [18] and prior work with hBN [17] , the results presented here demonstrated not only Type II but also Type I modes, which enabled the first exploration of such confinement in a Type I hyperbolic medium and provided the experimental investigation of their reciprocal spectral behaviours. Weaker resonances related to theoretically predicted [17] higher-order HP modes were identified experimentally in both Reststrahlen bands, and a more complete mode classification has been proposed. We report that both Reststrahlen bands supported two distinct series of HPs, which exhibited orthogonal requirements on the incident angle and polarization. This is the first description and experimental observation of these various series of HP modes. Future work may pursue the realization of hBN resonators of atomic dimensions [20] , [38] , [39] to achieve an ultimate confinement of these low-loss electromagnetic modes. Investigations into other polar van der Waal’s materials [27] such as MoS 2 , may further extend the spectral range where natural HMs are found [26] , [40] . These efforts may lead to the development of disruptive technologies such as the nanoscale equivalent of an optical fibre, due to the volume-bound confinement of sub-diffraction modes within hBN. Impact in areas such as enhanced molecular spectroscopy [41] , nanophotonic circuits [38] , tailored thermal emission sources [42] , [43] , flat optics [44] and super-resolution imaging [12] , [45] is also anticipated. hBN nanoresonator fabrication Flakes of hBN were exfoliated from crystals grown via the high-pressure/high-temperature method [46] , [47] and deposited on either 90-nm thick SiO 2 on doped n -type silicon, quartz or instrinsic silicon substrates using standard dicing tape. Using atomic force microscopy, the flakes of thicknesses 60–410 nm and spatial sizes sufficient for nanostructure array patterning (>50 μm on a side), were identified. The array patterns were defined using electron beam lithography and were patterned into a bilayer PMMA resist, with nanostructures ranging from 100 to 1,000 nm in diameter being fabricated, with the periodicity (centre-to-centre) being maintained at a 3:1 ratio with the designed diameter. A 30-nm thick aluminium film was deposited using thermal evaporation for the standard lift-off procedure and the hBN nanostructures were created by reactive ion etching in an inductively coupled CHF 3 /O 2 plasma (Oxford Instruments PlasmaLab) at a pressure of 10 mTorr, resulting in an etch rate of ~1 μm min −1 . The RF power applied to the plasma reactor and the substrate was 200 and 20 W, respectively. The CHF 3 /O 2 flow ratio (17.5/10 sccm) was optimized to increase the hBN-to-SiO 2 selectivity. The etch rates of the aluminium hard mask and SiO 2 substrates were determined to be insufficient for any significant etching to occur within this time. The aluminium hard mask was then removed via a standard TMAH (MICROPOSIT MF-319) wet chemical etchant. Optical characterization of hBN flakes and nanoresonators Mid-infrared reflectance measurements were undertaken using a Bruker Hyperion microscope coupled to a Bruker Vertex80v FTIR spectrometer. Three different objectives were used to obtain normal (ZnSe), off-normal ( × 36 Cassegrain) and grazing ( × 15 grazing incidence objective, GAO) incidence spectra from the nanostructures. The spectra were collected with a 2 cm −1 spectral resolution and spatial resolution defined by the internal adjustable aperture of the microscope that was set to the size of the specific array of interest. All measurements were performed in reference to a gold film. Derivation of optical constants for hBN Due to the large material anisotropy of hBN and the relatively small size of available flakes, optical constants were extracted using fits to reflection spectra from various thickness hBN flakes on BaF 2 substrates (see Supplementary Fig. 4 ). To derive the optical constants used in the electromagnetic modelling presented in Figs 2 , 4 and and the analytical calculations in Fig. 3 , the various spectra were fitted to calculations based on the standard transfer matrix approach, assuming the single-Lorentzian form of the principal dielectric tensor components [30] , [48] , [49] where a refers to either the transverse (a,b crystal plane) or z- (c crystal axis) axes, parameters ω LO , ω TO , ε ∞ and γ correspond to the LO and TO phonon frequencies, the high-frequency dielectric permittivity and the damping constant, respectively. The initial guess for these parameters was taken from Cai et al. [50] , while the BaF 2 optical response was taken from the optical constants provided in Palik’s compendium [51] . Numerical analysis To better understand the deeply sub-diffractional HP modes involved in these nanostructures, full-wave electrodynamic calculations were performed using the RF module of the finite-element package COMSOL. The anisotropic optical constants were extracted from the above-mentioned method and the geometry of the experimental nanostructures was determined from atomic force microscopy and scanning electron microscopy. The simulations were undertaken for the light incident at 0, 25 and 70° angles to match the illumination conditions of the ZnSe (0.08 NA), × 36 Cassegrain (0.52 NA) and GAO objectives of the Bruker FTIR microscopes described above. Analytical calculations for spheroidal resonators Although there is no analytical solution associated with complex geometries such as the conical nanoresonator shapes described here, analytical results for spheroidal nanoparticles can provide insight. The polariton modes of a spheroid of revolution with semi-axes a z and a x can be found by solving the anisotropic Laplace equation for the quasi-static scalar potential. The earliest complete solution of this eigenvalue problem known to us was reported in the early study [31] of magnetostatic waves in ferromagnets. More recently, the solution was independently rediscovered [32] in the context of polariton modes in ZnO quantum dots. The mode spectrum has been shown to satisfy the transcendental equation where and are the associated Legendre functions of the first and second kinds and parameters η 0 , η 1 are defined by For each azimuthal number m and orbital number l , equation (6) has several solutions that can in principle be labelled by another modal number r =1, 2,... This number corresponds to the number of radial oscillations in the scalar potential inside the spheroid. Following Walker [31] , one can show that in the case of hBN for non-zero m , the number of different radial modes is, respectively, p +1 and p for the upper and lower Reststrahlen band. Here p is the integer part of ( l − m )/2. For m =0, these numbers change to p and l−p , again for the upper (lower) band. Note that in the case of ZnO the total number of solutions is the same [32] ; however, the modes cannot be simply assigned to a particular band because unlike in hBN the two Reststrahlen bands of ZnO overlap spectrally. We solved equation (6) numerically using the standard library root-finding algorithms. The recurrence formulas for Legendre functions were used to compute these functions efficiently. From such calculations, we concluded that the best match to the experiment is obtained by assuming that all the observed modes belong to the r =1 family. Indeed, such modes have the largest dipole moment and so the largest coupling to the far-field radiation. The results of these calculations along with the corresponding resonant frequencies of the experimental results where available are provided in Fig. 3a,b of the main text for the and modes, respectively. Good agreement for the weaker modes was also found. How to cite this article: Caldwell, J. D. et al. Sub-diffractional, volume-confined polaritons in the natural hyperbolic material hexagonal boron nitride. Nat. Commun. 5:5221 doi: 10.1038/ncomms6221 (2014).